Ezh2 loss promotes development of myelodysplastic syndrome but attenuates its predisposition to leukaemic transformation Loss-of-function mutations of EZH2 , a catalytic component of polycomb repressive complex 2 (PRC2), are observed in ~\n10% of patients with myelodysplastic syndrome (MDS), but are rare in acute myeloid leukaemia (AML). Recent studies have shown that EZH2 mutations are often associated with RUNX1 mutations in MDS patients, although its pathological function remains to be addressed. Here we establish an MDS mouse model by transducing a RUNX1S291fs mutant into hematopoietic stem cells and subsequently deleting Ezh2 . Ezh2 loss significantly promotes RUNX1S291fs-induced MDS. Despite their compromised proliferative capacity of RUNX1S291fs/Ezh2 -null MDS cells, MDS bone marrow impairs normal hematopoietic cells via selectively activating inflammatory cytokine responses, thereby allowing propagation of MDS clones. In contrast, loss of Ezh2 prevents the transformation of AML via PRC1-mediated repression of Hoxa9 . These findings provide a comprehensive picture of how Ezh2 loss collaborates with RUNX1 mutants in the pathogenesis of MDS in both cell autonomous and non-autonomous manners. Recent genome sequencing studies have identified various mutations of epigenetic regulators in patients with myeloid malignancies such as myelodysplastic syndrome (MDS), myeloproliferative neoplasm (MPN) and acute myeloid leukaemia (AML) [1] , [2] , [3] . Epigenetic alterations are involved in the establishment of gene expression profiles associated with cancers, and the accumulation of genetic and epigenetic alterations promote tumorigenesis [4] , [5] . Among epigenetic regulators, polycomb-group (PcG) proteins have been implicated in many types of cancer. PcG proteins compose the polycomb repressive complexes 1 and 2 (PRC1 and PRC2), and function to repress the transcription of genes through monoubiquitination at H2AK119 (H2AK119ub1) and trimethylation at H3K27 (H3K27me3), respectively [6] , [7] . In the canonical pathway, PRC2 initiates gene silencing by catalysing H3K27me3 modification. PRC1 is then recruited to the target regions by binding to H3K27me3 through the CBX component of PRC1 (ref. 8) [8] , and then catalyses the monoubiquitination of H2AK119 to maintain gene silencing [9] . However, recent findings have shown that PRC1 can be recruited to target genes independently of H3K27me3 (refs 10 , 11 ). For example, the RUNX1 transcription factor has been shown to physically bind to Bmi1, a component of PRC1, and to recruit PRC1 in a PRC2-independent manner during the differentiation of megakaryocytes [12] . Since overexpression or gain-of-function mutations of EZH2 , a catalytic component of PRC2, are often found in carcinomas and lymphomas [2] , [13] , PcG genes have traditionally been characterized as oncogenes [5] . Specifically, overexpression of Ezh2 has been shown to lead to MPN [14] . We also reported that disease caused by MLL-AF9 requires Ezh2 for progression into AML in a mouse model [15] . These findings highlight the oncogenic function of EZH2 and are consistent with the findings that loss-of-function mutations of EZH2 are rare in de novo AML patients [2] , [16] . In contrast, ~\n10% of MDS patients harbour loss-of-function mutations in EZH2 (refs 16 , 17 ), excluding −7/7q− chromosome anomalies, which involves EZH2 located at 7q36. EZH2 mutations in MDS patients are associated with significantly worse prognosis, which is not due to AML transformation [1] , [18] . In addition, MDS patients without −7/7q− chromosome anomalies have reduced expression of EZH2 in CD34 + cells [19] , suggesting that EZH2 functions as a tumour suppressor in MDS. Indeed, we have recently shown that concurrent depletion of Ezh2 and Tet2 markedly accelerates the development of MDS and MDS/MPN in mice [20] . However, much remains unknown how EZH2 loss due to −7/7q− anomalies and loss-of-function mutations of EZH2 promotes the development of MDS. RUNX1 (also known as AML1 / CBFA2 ), a transcription factor critical for hematopoiesis, is frequently mutated (10–20%) in MDS patients and its mutations are significantly associated with −7/7q− chromosome anomalies [21] , [22] . Recent studies have demonstrated that RUNX1 mutations are one of several alterations significantly associated with EZH2 mutations in MDS patients and that both mutations independently predict poor prognosis [1] , [18] , [23] . RUNX1S291fs mutant retains a DNA binding domain but lacks a transactivation domain in the carboxy terminus [22] . It has been demonstrated that transduction of RUNX1S291fs into bone marrow (BM) progenitor cells is sufficient to induce MDS and AML following MDS (MDS/AML) in vivo , although it takes a long latency [24] . Given these findings, we set about to understand the molecular mechanism underlying the pathogenesis of MDS. We established a novel MDS mouse model utilizing Ezh2 -dificient hematopoietic stem cells (HSCs) and the RUNX1S291fs mutant. In this study, we found that Ezh2 loss significantly promoted the transformation of HSCs expressing the RUNX1S291fs mutant into MDS cells in vivo . Of note, RUNX1S291fs/Ezh2- null hematopoietic stem/progenitor cells (HSPCs) did not activate the expression of potent leukaemic oncogenes such as Hoxa9 and Mecom/Evi1 and showed compromised proliferative capacity, consistent with the impaired proliferative capacity of human MDS HSPCs [25] . We also found HOXA9 expression to be closely repressed in CD34 + HSPCs from the early stage MDS patients. While deregulation of HSC function is an important step for the development of myeloid malignancies [26] , recent studies indicate that BM microenvironment is another critical factor for the development of myeloid malignancies including MDS [27] , [28] . Chronic myeloid leukaemia (CML) cells also affect the function of BM microenvironment to impair normal hematopoiesis and support CML stem cell function [29] , [30] . Here, despite the compromised proliferative capacity, RUNX1S291fs/Ezh2- null MDS cells outcompete residing wild-type (WT) cells in the MDS BM by activating inflammatory cytokine responses, including the interleukin-6 (IL-6) pathway, which have been shown to impair normal HSCs in vivo . Thus, the MDS BM environment negatively impacts normal HSCs, but not the MDS cells, thereby allowing propagation of MDS clones. Finally, we demonstrate that Ezh2 loss is incompatible with the leukaemic transformation of MDS clones partly due to the inactivation of Hoxa9 on loss of Ezh2. Ezh2 loss promotes RUNX1 mutant-induced MDS Given that RUNX1 mutations are identified in ~\n30% of MDS patients harbouring EZH2 loss-of-function mutations [1] , [18] , [23] , we examined how Ezh2 loss and RUNX1 mutants collaborate in the development of MDS in vivo . To do so, we transduced a RUNX1S291fs-IRES-GFP or a control empty-IRES-GFP retroviral construct into either Cre-ERT ; Ezh2 wt/wt or Cre-ERT ; Ezh2 flox/flox (CD45.2 + ) CD34 − Lin − Sca1 − c-Kit + (LSK) HSCs ( Fig. 1a ). The transduced cells were transplanted into lethally irradiated CD45.1 + -recipient mice together with radioprotective CD45.1 + BM cells ( Fig. 1a ). The CD45.2 + GFP + -transduced cells successfully engrafted and established significant levels of chimerism in the peripheral blood (PB) at 1 month post transplantation ( Supplementary Fig. 1 ), and expressed the RUNX1S291fs protein ( Fig. 1b ). We then proceeded to activate Cre-ERT recombinase at 6 weeks post transplantation by intraperitoneal injection of tamoxifen ( Fig. 1a ). We hereafter refer to the recipient mice reconstituted with Empty/Ezh2 wt/wt , Empty/Ezh2 Δ/Δ , RUNX1S291fs/Ezh2 wt/wt and RUNX1S291fs/Ezh2 Δ/Δ -transduced HSCs as WT, Ezh2 Δ/Δ , Rx291 and Rx291/Ezh2 Δ/Δ mice, respectively ( Fig. 1a ). We confirmed successful deletions of Ezh2 ( Supplementary Fig. 2 ), and markedly reduced the levels of H3K27me3 in CD45.2 + GFP + Lin − c-Kit + BM cells isolated from Ezh2 Δ/Δ and Rx291/Ezh2 Δ/Δ mice ( Fig. 1b ). Although levels of RUNX1S291fs transcripts were comparable between Rx291 and Rx291/Ezh2 Δ/Δ cells ( Supplementary Fig. 3 ), level of RUNX1S291fs protein was much higher in Rx291/Ezh2 Δ/Δ cells ( Fig. 1b ), suggesting that Ezh2 loss somehow impacts the levels of RUNX1S291fs protein post transcriptionally. 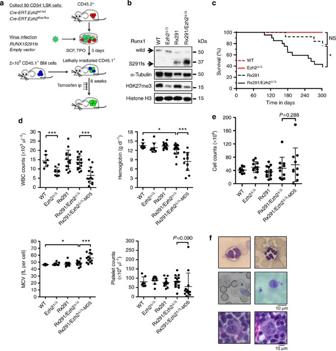Figure 1: Ezh2 loss promotes formation of RUNX1S291fs mutant-induced MDS. (a) Experimental scheme of our model mouse utilizingRUNX1S291fsmutant andEzh2conditional knockout HSCs. (b) Successful transductions of RUNX1S291fs protein and levels of H3K27me3 in Lin−c-Kit+cells detected by western blotting. α-Tubulin and histone H3 were detected as loading controls. (c) Significantly shorter median survival of Rx291/Ezh2Δ/Δmice (n=21) compared with Rx291 mice (n=18) (262 days versus undetermined,P=0.038 by Log-rank test). (d) Complete blood cell counts of WT (n=7), Ezh2Δ/Δ(n=9), Rx291 (n=15) and Rx291/Ezh2Δ/Δ(n=17) mice at 4 months post transplantation (pre-MDS stage) and moribund Rx291/Ezh2Δ/Δ-MDS mice (n=13). Rx291/Ezh2Δ/Δmice showed reduced hemoglobin levels and increased mean corpuscular volume (MCV) compared with WT mice (12.4±1.7 versus 13.6±0.9,P=0.047 and 48.7±3.2 versus 46.5±0.7,P=0.048 by Student’st-test, respectively). Moribund Rx291/Ezh2Δ/Δ-MDS mice showed significant leukopenia and macrocytic anaemia compared with Rx291/Ezh2Δ/Δmice at 4 months post transplantation (pre-MDS stage). Scale bars and asterisks show mean±s.d., *P<0.05, **P<0.01, and ***P<0.001 by Student’st-test. (e) BM cell counts (from bilateral femurs and tibiae) in WT, Ezh2Δ/Δ, Rx291 and Rx291/Ezh2Δ/Δmice at 4 months post transplantation (pre-MDS stage) and moribund Rx291/Ezh2Δ/Δ-MDS mice. Comparable cell counts were seen in Rx291/Ezh2Δ/Δ(n=10) and Rx291/Ezh2Δ/Δ-MDS mice (n=10). Scale bars show mean±s.d.P-value was determined by Student’st-test. (f) Appearance of dysplastic blood cells in Rx291/Ezh2Δ/Δ-MDS mice observed by May–Grüenwald Giemsa staining. Pseudo-Pelger–Huët cell (PB), hypersegmented neutrophil (PB), a giant platelet (PB), hypolobated megakaryocytes (BM) and nucleated red blood cells (PB) are depicted (clockwise from the upper left picture). Scale bars, 10 μm. ip, intraperitoneal. Figure 1: Ezh2 loss promotes formation of RUNX1S291fs mutant-induced MDS. ( a ) Experimental scheme of our model mouse utilizing RUNX1S291fs mutant and Ezh2 conditional knockout HSCs. ( b ) Successful transductions of RUNX1S291fs protein and levels of H3K27me3 in Lin − c-Kit + cells detected by western blotting. α-Tubulin and histone H3 were detected as loading controls. ( c ) Significantly shorter median survival of Rx291/Ezh2 Δ/Δ mice ( n =21) compared with Rx291 mice ( n =18) (262 days versus undetermined, P =0.038 by Log-rank test). ( d ) Complete blood cell counts of WT ( n =7), Ezh2 Δ/Δ ( n =9), Rx291 ( n =15) and Rx291/Ezh2 Δ/Δ ( n =17) mice at 4 months post transplantation (pre-MDS stage) and moribund Rx291/Ezh2 Δ/Δ -MDS mice ( n =13). Rx291/Ezh2 Δ/Δ mice showed reduced hemoglobin levels and increased mean corpuscular volume (MCV) compared with WT mice (12.4±1.7 versus 13.6±0.9, P =0.047 and 48.7±3.2 versus 46.5±0.7, P =0.048 by Student’s t -test, respectively). Moribund Rx291/Ezh2 Δ/Δ -MDS mice showed significant leukopenia and macrocytic anaemia compared with Rx291/Ezh2 Δ/Δ mice at 4 months post transplantation (pre-MDS stage). Scale bars and asterisks show mean±s.d., * P <0.05, ** P <0.01, and *** P <0.001 by Student’s t -test. ( e ) BM cell counts (from bilateral femurs and tibiae) in WT, Ezh2 Δ/Δ , Rx291 and Rx291/Ezh2 Δ/Δ mice at 4 months post transplantation (pre-MDS stage) and moribund Rx291/Ezh2 Δ/Δ -MDS mice. Comparable cell counts were seen in Rx291/Ezh2 Δ/Δ ( n =10) and Rx291/Ezh2 Δ/Δ -MDS mice ( n =10). Scale bars show mean±s.d. P -value was determined by Student’s t -test. ( f ) Appearance of dysplastic blood cells in Rx291/Ezh2 Δ/Δ -MDS mice observed by May–Grüenwald Giemsa staining. Pseudo-Pelger–Huët cell (PB), hypersegmented neutrophil (PB), a giant platelet (PB), hypolobated megakaryocytes (BM) and nucleated red blood cells (PB) are depicted (clockwise from the upper left picture). Scale bars, 10 μm. ip, intraperitoneal. Full size image We first examined whether Ezh2 loss contributes to the development of MDS in recipient mice. While WT mice ( n =9) and Ezh2 Δ/Δ mice ( n =9) did not develop lethal haematological malignancies within 10 months post transplantation, Rx291 and Rx291/Ezh2 Δ/Δ mice developed MDS. Rx291/Ezh2 Δ/Δ mice showed a significantly shorter median survival than Rx291 mice did (262 days versus undetermined, P =0.038) ( Fig. 1c ), indicating that Ezh2 loss facilitates disease progression. Although Rx291/Ezh2 Δ/Δ mice did not show any significant changes in the peripheral complete blood counts until 3 months post transplantation, they started to show reduced haemoglobin levels and increased mean corpuscular volume compared with WT mice at 4 months post transplantation ( Fig. 1d ). Ezh2 Δ/Δ mice showed a significant leukopenia, in part due to impaired lymphopoiesis as previously reported [31] , [32] . While only 2 out of 18 Rx291 mice developed MDS within 10 months post transplantation, 13 out of 21 Rx291/Ezh2 Δ/Δ mice developed MDS including one MDS/myeloid leukaemia (MDS/ML) showing very slow disease progression that did not match the criteria of ‘acute’ leukaemia in the Bethesda proposal ( Fig. 1c and Supplementary Table 1 ) [33] . Moribund Rx291/Ezh2 Δ/Δ mice with MDS including MDS/ML (Rx291/Ezh2 Δ/Δ -MDS mice) showed significant leukopenia and macrocytic anaemia (anaemia with increased mean corpuscular volume) compared with Rx291/Ezh2 Δ/Δ mice at pre-MDS stage ( Fig. 1d ). BM cellularity was variable among Rx291/Ezh2 Δ/Δ -MDS mice, implying heterogeneous disease status ( Fig. 1e ). Rx291/Ezh2 Δ/Δ -MDS mice also showed dysplastic cells characteristic of human MDS such as pseudo-Pelger–Huët cells, hypersegmented neutrophils, nucleated red blood cells, giant platelets and hypolobated megakaryocytes ( Fig. 1f ) [34] . Thus, our model mice present with leukopenia, anaemia and multilineage dysplasia, phenotypically recapitulating human MDS. In addition, we also confirmed that Ezh2 loss significantly promotes the development of MDS induced by RUNX1D171N , another RUNX1 mutant defective in DNA binding, although RUNX1D171N -mutant cells exhibited a relatively long latency (D171N/Ezh2 Δ/Δ ( n =5) versus D171N/Ezh2 wt/wt ( n =7); 353 days versus undetermined, P =0.0133 by Log-rank test). These findings indicate that Ezh2 can function as a tumour suppressor in MDS, especially in the presence of RUNX1 mutants. Ezh2 loss provokes ineffective hematopoiesis MDS patients show ineffective hematopoiesis characterized by impaired differentiation and enhanced apoptosis of BM cells that leads to cytopenia [35] . To evaluate hematopoiesis in Rx291/Ezh2 Δ/Δ -MDS mice, we first examined chimerism of CD45.2 + GFP + cells in HSCs (CD34 − LSK), HSPCs (LSK) and Lin − c-Kit + Sca1 − (LK) myeloid progenitor cells in the BM and myeloid cells and lymphoid cells in the PB. While Ezh2 Δ/Δ and Rx291 mice showed comparable chimerism of CD45.2 + GFP + mutant cells in both BM and PB, both Rx291/Ezh2 Δ/Δ (at pre-MDS stage) and Rx291/Ezh2 Δ/Δ -MDS (at terminal stage) mice showed higher chimerism in BM HSCs and HSPCs, but contradictory lower chimerism in PB ( Fig. 2a ), due to impaired production of Mac1 + myeloid cells, CD4 + /CD8 + T cells and B220 + B cells ( Fig. 2b ). These findings indicate that on deletion of Ezh2 , RUNX1S291fs -expressing HSCs acquire a competitive disadvantage in terms of their ability to generate PB cells. 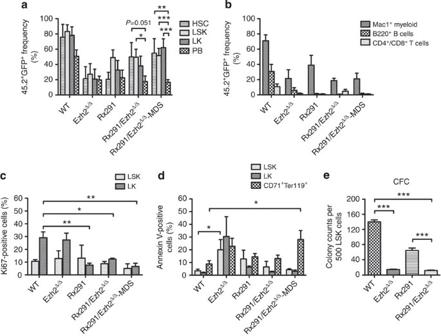Figure 2: Ezh2 loss confers a competitive disadvantage to RUNX1S291fs-expressing HSPCs. (a) Chimerism of CD45.2+GFP+cells in HSCs, LSK cells and LK cells in the BM and PB cells in WT, Ezh2Δ/Δ, Rx291 and Rx291/Ezh2Δ/Δmice at 4 months post transplantation (pre-MDS stage) (n=4–6) and moribund Rx291/Ezh2Δ/Δ-MDS mice (n=12). Scale bars and asterisks show mean±s.d. and *P<0.05, **P<0.01 and ***P<0.001 by Student’st-test. (b) Chimerism of CD45.2+GFP+of Mac1+myeloid cells, B220+B cells and CD4+/CD8+T cells in the PB analysed ina. Scale bars show mean±s.d. (c) Proliferative capacity examined with Ki67 in (CD45.2+GFP+) LSK and LK cells in WT, Ezh2Δ/Δ, Rx291 and Rx291/Ezh2Δ/Δmice at 4 months post transplantation (n=3–5) and moribund Rx291/Ezh2Δ/Δ-MDS mice (n=3). Scale bars and asterisks show mean±s.e.m., *P<0.05 and **P<0.01 by Student’st-test. (d) Enhanced apoptosis in CD71+Ter119+Rx291/Ezh2Δ/Δ-MDS erythroblasts but not in MDS LSK/LK stem and progenitor cells in WT, Ezh2Δ/Δ, Rx291 and Rx291/Ezh2Δ/Δmice at 4 months post transplantation (n=3–6) and moribund Rx291/Ezh2Δ/Δ-MDS mice (n=4). Scale bars and asterisks show mean±s.e.m. and *P<0.05 by Student’st-test. (e) Clonogenic capacity of 500 (CD45.2+GFP+) LSK cells isolated from WT, Ezh2Δ/Δ, Rx291 and Rx291/Ezh2Δ/Δmice at 4 months post transplantation (n=3). Scale bars and asterisk show mean±s.e.m. and ***P<0.001 by Student’st-test. Figure 2: Ezh2 loss confers a competitive disadvantage to RUNX1S291fs-expressing HSPCs. ( a ) Chimerism of CD45.2 + GFP + cells in HSCs, LSK cells and LK cells in the BM and PB cells in WT, Ezh2 Δ/Δ , Rx291 and Rx291/Ezh2 Δ/Δ mice at 4 months post transplantation (pre-MDS stage) ( n =4–6) and moribund Rx291/Ezh2 Δ/Δ -MDS mice ( n =12). Scale bars and asterisks show mean±s.d. and * P <0.05, ** P <0.01 and *** P <0.001 by Student’s t -test. ( b ) Chimerism of CD45.2 + GFP + of Mac1 + myeloid cells, B220 + B cells and CD4 + /CD8 + T cells in the PB analysed in a . Scale bars show mean±s.d. ( c ) Proliferative capacity examined with Ki67 in (CD45.2 + GFP + ) LSK and LK cells in WT, Ezh2 Δ/Δ , Rx291 and Rx291/Ezh2 Δ/Δ mice at 4 months post transplantation ( n =3–5) and moribund Rx291/Ezh2 Δ/Δ -MDS mice ( n =3). Scale bars and asterisks show mean±s.e.m., * P <0.05 and ** P <0.01 by Student’s t -test. ( d ) Enhanced apoptosis in CD71 + Ter119 + Rx291/Ezh2 Δ/Δ -MDS erythroblasts but not in MDS LSK/LK stem and progenitor cells in WT, Ezh2 Δ/Δ , Rx291 and Rx291/Ezh2 Δ/Δ mice at 4 months post transplantation ( n =3–6) and moribund Rx291/Ezh2 Δ/Δ -MDS mice ( n =4). Scale bars and asterisks show mean±s.e.m. and * P <0.05 by Student’s t -test. ( e ) Clonogenic capacity of 500 (CD45.2 + GFP + ) LSK cells isolated from WT, Ezh2 Δ/Δ , Rx291 and Rx291/Ezh2 Δ/Δ mice at 4 months post transplantation ( n =3). Scale bars and asterisk show mean±s.e.m. and *** P <0.001 by Student’s t -test. Full size image We then examined proliferative capacity of stem/myeloid progenitor cells by staining with Ki67, a marker for cellular proliferation. Transduction of RUNX1S291fs appeared to reduce Ki67 + frequencies in LK myeloid progenitor cells and in LSK cells, and this trend was even more evident in LK cells in Rx291/Ezh2 Δ/Δ -MDS mice ( Fig. 2c ). Thus, the proliferative capacity of Rx291/Ezh2 Δ/Δ cells was attenuated during the development of MDS, especially in myeloid progenitor cells. As Rx291/Ezh2 Δ/Δ -MDS mice also showed anaemia, we next examined the apoptosis of BM cells by Annexin V staining. Ezh2 Δ/Δ mice showed enhanced apoptosis especially in LSK cells ( Fig. 2d ). Rx291/Ezh2 Δ/Δ -MDS mice showed enhanced apoptosis in (CD45.2 + GFP + ) CD71 + Ter119 + erythroblasts, but not in LK and LSK cells, compared with WT mice ( Fig. 2d ), implying that RUNX1S291fs mutant suppressed the Ezh2 loss-induced apoptosis in LSK cells. Previous studies have shown that the in vitro colony-forming capacity of HSPCs isolated from MDS patients and MDS mouse models is impaired [25] , [36] . Consistent with these findings, we found that Rx291/Ezh2 Δ/Δ LSK cells generated significantly fewer colonies in vitro than WT and Rx291 LSK cells ( Fig. 2e ). Taken together, the impaired proliferative capacity of myeloid progenitor cells and enhanced apoptosis in erythroblasts may account for the cytopenia observed in Rx291/Ezh2 Δ/Δ -MDS mice. Thus, our mouse model also recapitulates ineffective hematopoiesis, one of the pathological features of MDS. Ezh2 loss promotes initiation and propagation of MDS Since Rx291/Ezh2 Δ/Δ HSPCs were capable of potent induction of MDS despite their impaired proliferative capacity and competitive disadvantage in generating PB cells, we examined the repopulating capacity of Rx291 and Rx291/Ezh2 Δ/Δ cells in detail by employing a limiting dilution transplantation assay utilizing 2 × 10 4 , 2 × 10 3 and 200 CD45.2 + GFP + Lin − c-Kit + cells isolated from the primary Rx291 and Rx291/Ezh2 Δ/Δ mice at pre-MDS stage together with 2 × 10 5 competitor CD45.1 + BM cells. We considered the recipient mice showing chimerism of CD45.2 + GFP + cells >1% in PB at 4 months post transplantation as positively repopulated mice. Rx291 Lin − c-Kit + cells did not repopulate any mice in any experiments, whereas Rx291/Ezh2 Δ/Δ Lin − c-Kit + cells at a dose of 2 × 10 4 cells positively repopulated two out of seven recipient mice, allowing estimation of the frequency of repopulating cells to be between 1 in 259,626 and 1 in 16,318 Lin − c-Kit + cells (95% confidence interval)( Table 1 ). Notably, these Rx291/Ezh2 Δ/Δ cells repopulated in the positive mice outcompeted the WT competitor cells in the BM ( Fig. 3a ), and induced MDS by 6 months post transplantation as indicated by dysplastic neutrophils, nucleated red blood cells, hypolobated megakaryocytes in the BM ( Fig. 3b ), as well as mild macrocytic anaemia. Thus, loss of Ezh2 promotes the expansion of MDS-initiating cells in HSPCs expressing RUNX1S291fs at the ‘pre-MDS phase’. Table 1 Frequency of repopulating cells in RUNX1S291fs-induced cells. 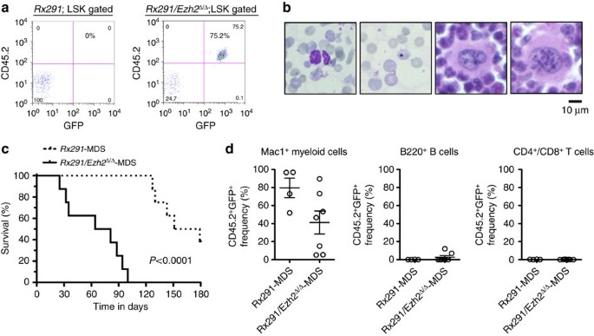Figure 3: Ezh2 loss promotes initiation and propagation of RUNX1S291fs-induced MDS. (a) Representative flow cytometric profiles of LSK cells in recipient mice infused with 2 × 104Rx291orRx291/Ezh2Δ/ΔLin−c-Kit+cells at 6 months post transplantation. Proportion of CD45.2+GFP+cells within LSK cells was indicated (%). (b) Dysplastic neutrophils, red blood cells and megakaryocytes in the BM of the positively repopulated recipient mice inathat developed MDS. Scale bar, 10 μm. (c) Significantly shorter median survival of recipients ofRx291/Ezh2Δ/Δ-MDS cells (n=8), compared with those ofRx291-MDS cells (n=8)(72.5 days versus 165 days;P<0.0001 by Log-rank test). Lethally irradiated recipient mice were infused with 1 × 106CD45.2+GFP+RUNX1S291fs-expressing BM cells isolated from Rx291-MDS mice or Rx291/Ezh2Δ/Δ-MDS mice together with 2 × 105competitor CD45.1+BM cells. (d) Chimerism of CD45.2+GFP+cells in Mac1+myeloid cells, B220+B cells and CD4+/CD8+T cells in the PB in Rx291-MDS (n=4) and Rx291/Ezh2Δ/Δ-MDS recipient mice (n=7) at the advanced MDS stage. Scale bars show mean±s.e.m. Full size table Figure 3: Ezh2 loss promotes initiation and propagation of RUNX1S291fs-induced MDS. ( a ) Representative flow cytometric profiles of LSK cells in recipient mice infused with 2 × 10 4 Rx291 or Rx291/Ezh2 Δ/Δ Lin − c-Kit + cells at 6 months post transplantation. Proportion of CD45.2 + GFP + cells within LSK cells was indicated (%). ( b ) Dysplastic neutrophils, red blood cells and megakaryocytes in the BM of the positively repopulated recipient mice in a that developed MDS. Scale bar, 10 μm. ( c ) Significantly shorter median survival of recipients of Rx291/Ezh2 Δ/Δ -MDS cells ( n =8), compared with those of Rx291 -MDS cells ( n =8)(72.5 days versus 165 days; P <0.0001 by Log-rank test). Lethally irradiated recipient mice were infused with 1 × 10 6 CD45.2 + GFP + RUNX1S291fs-expressing BM cells isolated from Rx291-MDS mice or Rx291/Ezh2 Δ/Δ -MDS mice together with 2 × 10 5 competitor CD45.1 + BM cells. ( d ) Chimerism of CD45.2 + GFP + cells in Mac1 + myeloid cells, B220 + B cells and CD4 + /CD8 + T cells in the PB in Rx291-MDS ( n =4) and Rx291/Ezh2 Δ/Δ -MDS recipient mice ( n =7) at the advanced MDS stage. Scale bars show mean±s.e.m. Full size image Since both Rx291 and Rx291/Ezh2 Δ/Δ mice developed MDS albeit with different latencies ( Fig. 1c ), we next investigated whether RUNX1S291fs -induced MDS cells could propagate in secondary recipients in the absence of Ezh2. We transplanted 1 × 10 6 CD45.2 + GFP + RUNX1S291fs-expressing BM cells isolated from Rx291-MDS and Rx291/Ezh2 Δ/Δ -MDS mice independently into lethally irradiated CD45.1 + recipient mice together with 2 × 10 5 CD45.1 + BM cells. We found that all secondary recipients infused with Rx291/Ezh2 Δ/Δ -MDS cells died from MDS within 100 days, whereas those with Rx291 -MDS cells took much longer to develop lethal MDS (median survival, 72.5 days versus 165 days; P <0.0001) ( Fig. 3c ). Furthermore, production of peripheral myeloid cells by Rx291/Ezh2 Δ/Δ -MDS cells appeared to be less efficient compared with Rx291 -MDS cells at the advanced MDS stage ( Fig. 3d ), again suggesting ineffective hematopoiesis by Rx291/Ezh2 Δ/Δ -MDS cells. These findings indicate that Ezh2 loss promotes both initiation and propagation of RUNX1S291fs -induced MDS. Ezh2 target genes were repressed in Ezh2 -null MDS HSPCs To understand how Ezh2 loss promotes RUNX1S291fs-induced MDS, we began to investigate gene expression profiles in CD45.2 + GFP + LSK cells isolated from WT, Ezh2 Δ/Δ , Rx291, Rx291/Ezh2 Δ/Δ (at 4 months post transplantation), and two Rx291/Ezh2 Δ/Δ -MDS mice (MDS and MDS/ML). Since Ezh2 functions to repress transcription via H3K27me3 modification, its absence is supposed to activate transcription of its target genes. As expected, gene set enrichment analysis (GSEA) revealed that Ezh2 Δ/Δ LSK cells significantly de-repressed canonical Ezh2 target genes ( Table 2 and Supplementary Fig. 4 ), defined in murine ES cells (GSE15388) [37] . However, Ezh2 targets were negatively enriched in both Rx291/Ezh2 Δ/Δ -MDS and MDS/ML LSK cells, compared with WT LSK cells ( Table 2 ). Repression of Ezh2 target genes was also evident when we compared Rx291/Ezh2 Δ/Δ -MDS LSK cells to Rx291/Ezh2 Δ/Δ LSK cells at the pre-MDS phase ( Fig. 4a ), indicating that Ezh2 targets underwent transcriptional repression during the development of MDS despite the absence of Ezh2. This finding is similar to our previous observations on MDS developed in Tet2 KD/KD Ezh2 Δ/Δ mice compound for Tet2 hypomorphic gene trap ( Tet2 KD/KD ) and conditional deletion of Ezh2 , where repression of Ezh2 target genes was attributed to the compensatory function of Ezh1, another catalytic component of PRC2 (ref. 20) [20] . Table 2 GSEA for Ezh2 targets and AML-related targets. 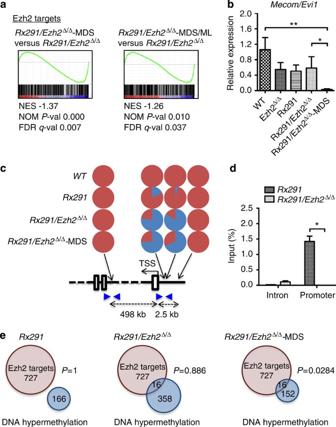Figure 4:RUNX1S291fs/Ezh2-null MDS HSPCs represses expression of Ezh2 target genes. (a) Gene set enrichment plots for the canonical Ezh2 target gene set comparingRx291/Ezh2Δ/Δ-MDS (left panel) andRx291/Ezh2Δ/Δ-MDS/ML (right panel) LSK cells withRx291/Ezh2Δ/ΔLSK cells at pre-MDS stage. (b) Quantitative RT–PCR analysis of the expression ofMecom/Evi1in CD45.2+GFP+LSK cells from in WT, Ezh2Δ/Δ, Rx291 and Rx291/Ezh2Δ/Δmice at 4 months post transplantation (pre-MDS stage) and moribund Rx291/Ezh2Δ/Δ-MDS mice (n=4–5). Scale bars and asterisks show mean±s.e.m., *P<0.05 and **P<0.01 by Mann–WhitneyU-test. (c) DNA methylation status at promoter and intron regions ofMecom/Evi1detected by RRBS in LSK cells from WT, Rx291 and Rx291/Ezh2Δ/Δmice at 4 months post transplantation (pre-MDS stage) and from moribund Rx291/Ezh2Δ/Δ-MDS mouse. The proportion of methylated (in blue) and non-methylated (in red) cytosines at mm9 position chr3:29911333 (downstream intron), chr3:30409294 and 30409295 (promoter) and chr3:30407526 (upstream) are depicted in circles. Blue arrowheads indicate regions amplified by ChIP–QPCR ind. (d) The levels of H3K27me3 at the promoter and intron regions ofMecom/Evi1inRx291andRx291/Ezh2Δ/ΔLSK cells as detected by ChIP–QPCR. The relative amounts of immunoprecipitated DNA are depicted as a percentage of input DNA. Scale bars and asterisks show mean±s.e.m. (n=4), and *P<0.05 by Mann–WhitneyU-test. (e) Venn diagrams of overlaps between canonical Ezh2 target genes and DNA hypermethylated genes inRx291,Rx291/Ezh2Δ/ΔorRx291/Ezh2Δ/Δ-MDS LSK cells. Total number of genes was 13146.P-value of intersection was determined by usingRcode. Full size table Figure 4: RUNX1S291fs/Ezh2 -null MDS HSPCs represses expression of Ezh2 target genes. ( a ) Gene set enrichment plots for the canonical Ezh2 target gene set comparing Rx291/Ezh2 Δ/Δ -MDS (left panel) and Rx291/Ezh2 Δ/Δ -MDS/ML (right panel) LSK cells with Rx291/Ezh2 Δ/Δ LSK cells at pre-MDS stage. ( b ) Quantitative RT–PCR analysis of the expression of Mecom/Evi1 in CD45.2 + GFP + LSK cells from in WT, Ezh2 Δ/Δ , Rx291 and Rx291/Ezh2 Δ/Δ mice at 4 months post transplantation (pre-MDS stage) and moribund Rx291/Ezh2 Δ/Δ -MDS mice ( n =4–5). Scale bars and asterisks show mean±s.e.m., * P <0.05 and ** P <0.01 by Mann–Whitney U -test. ( c ) DNA methylation status at promoter and intron regions of Mecom/Evi1 detected by RRBS in LSK cells from WT, Rx291 and Rx291/Ezh2 Δ/Δ mice at 4 months post transplantation (pre-MDS stage) and from moribund Rx291/Ezh2 Δ/Δ -MDS mouse. The proportion of methylated (in blue) and non-methylated (in red) cytosines at mm9 position chr3:29911333 (downstream intron), chr3:30409294 and 30409295 (promoter) and chr3:30407526 (upstream) are depicted in circles. Blue arrowheads indicate regions amplified by ChIP–QPCR in d . ( d ) The levels of H3K27me3 at the promoter and intron regions of Mecom/Evi1 in Rx291 and Rx291/Ezh2 Δ/Δ LSK cells as detected by ChIP–QPCR. The relative amounts of immunoprecipitated DNA are depicted as a percentage of input DNA. Scale bars and asterisks show mean±s.e.m. ( n =4), and * P <0.05 by Mann–Whitney U -test. ( e ) Venn diagrams of overlaps between canonical Ezh2 target genes and DNA hypermethylated genes in Rx291 , Rx291/Ezh2 Δ/Δ or Rx291/Ezh2 Δ/Δ -MDS LSK cells. Total number of genes was 13146. P -value of intersection was determined by using R code. Full size image We next examined the expression of ‘HSC fingerprint genes’, a gene set specific to HSCs defined by extensive microarray analyses [38] . RUNX1S291fs repressed expression of ‘HSC fingerprint genes’ and this trend was more evident in Rx291/Ezh2 Δ/Δ and Rx291/Ezh2 Δ/Δ -MDS LSK cells ( Table 2 and Supplementary Fig. 4 ). RT–PCR analysis confirmed downregulation of ‘HSC fingerprint genes’ such as Mecom/Evi1 ( Fig. 4b ), which is a well-known oncogene that plays a critical role for both HSCs and AML [39] . Of note, expression of Mecom/Evi1 became further repressed in Rx291/Ezh2 Δ/Δ -MDS LSK cells, compared with Rx291/Ezh2 Δ/Δ LSK cells ( Fig. 4b ), suggesting that some epigenetic events took place during the disease progression at the Mecom/Evi1 region. Promoter DNA hypermethylation is one of the most well-known epigenetic events that propagates during tumour development [40] . We postulated that promoter DNA hypermethylation might also be involved in the transcriptional repression of Ezh2 targets and ‘HSC fingerprint genes’ in the absence of Ezh2. To evaluate promoter DNA hypermethylation in LSK cells, we performed reduced representation bisulphite sequencing (RRBS). Compared with WT (CD45.2 + GFP + ) LSK cells, we found 232, 512 and 204 hypermethylated promoters in Rx291 , Rx291/Ezh2 Δ/Δ and Rx291/Ezh2 Δ/Δ -MDS (CD45.2 + GFP + ) LSK cells, respectively (annotated gene lists are shown in Supplementary Data 1 ). Notably, the promoter regions of Mecom/Evi1 acquired DNA hypermethylation in Rx291/Ezh2 Δ/Δ and Rx291/Ezh2 Δ/Δ -MDS LSK cells, but not in Rx291 LSK cells, ( Fig. 4c ). This hypermethylation was coincided loss of H3K27me3 at the promoter on deletion of Ezh2 ( Fig. 4d ). These findings imply that Mecom/Evi1 is a direct target of Ezh2 in this context. We next examined the correlation between canonical Ezh2 targets in ES cells and genes that underwent DNA hypermethylation identified in this study. Some DNA hypermethylated genes overlapped with the canonical Ezh2 targets in Rx291/Ezh2 Δ/Δ LSK cells (16 out of 374 genes, P =0.886) and Rx291/Ezh2 Δ/Δ -MDS LSK cells (16 out of 168 genes, P =0.0284), but not in Rx291 LSK cells ( Fig. 4e ), and appeared to be developmental regulators of hematopoietic and non-hematopoietic lineages (for example, Mecom/Evi1 , Pdx1 and Hand1 ) ( Supplementary Table 2 ), suggesting that aberrant promoter DNA hypermethylation is an alternative epigenetic mechanism that represses Ezh2 targets in the absence of Ezh2. RUNX1S291fs/Ezh2 -null cells compromise normal HSPCs function Although Rx291/Ezh2 Δ/Δ HSPCs did not show enhanced proliferative capacity, Rx291/Ezh2 Δ/Δ cells were able to induce MDS at a lower dose compared with Rx291 cells. However, the mechanism by which the Rx291/Ezh2 Δ/Δ cells outcompeted WT cells was unclear. Given that BM environment is critical for the development of myeloid malignancies [27] , [28] , we postulated that CD45.1 + WT cells in Rx291/Ezh2 Δ/Δ mice might be depleted via indirect mechanisms associated with MDS. We did not see obvious differences in the frequencies of phenotypic LSK HSPCs in CD45.1 + cells between Rx291 and Rx291/Ezh2 Δ/Δ mice ( n =4; mean±s.d. 0.0495±0.0668% versus 0.0661±0.0449%; P =0.694 by Student’s t -test). However, colony-forming cells were significantly reduced in CD45.1 + WT LSK cells isolated from Rx291/Ezh2 Δ/Δ mice, compared with those from Rx291 mice and the primary WT LSK cells ( Supplementary Fig. 5 ). To assess the repopulating capacity of CD45.1 + WT HSPCs in vivo , 2 × 10 5 CD45.1 + WT BM cells isolated from Rx291 mice or Rx291/Ezh2 Δ/Δ mice were transplanted with an equal number of 8-week-old CD45.2 + competitor BM cells into lethally irradiated CD45.2 + -recipient mice ( Fig. 5a ). CD45.1 + cells from Rx291/Ezh2 Δ/Δ mice scarcely contributed to LSK cells in BM and mature hematopoietic cells in PB at 4 months post competitive transplantation, whereas CD45.1 + cells from Rx291 mice reconstituted hematopoiesis efficiently ( Fig. 5b ). These findings indicate that the function of WT HSPCs in Rx291/Ezh2 Δ/Δ mice is markedly impaired. To understand the underlying mechanism, we examined gene expression profiles of CD45.1 + LSK cells isolated from Rx291 and Rx291/Ezh2 Δ/Δ mice. Recent studies indicated that inflammatory cytokines are critical factors to regulate normal HSCs under both homeostatic and stress conditions such as infection [41] , [42] . GSEA revealed upregulation of genes related to interferon-γ and IL-6 pathways in CD45.1 + WT LSK cells from Rx291/Ezh2 Δ/Δ mice compared with WT LSK cells from WT mice ( Supplementary Table 3 ), suggesting activation of inflammatory cytokine responses in residual normal HSPCs in Rx291/Ezh2 Δ/Δ mice. Furthermore, upregulation of IL-6 and tumor necrosis factor alpha (TNFα) pathways was evident when we compared CD45.1 + WT LSK cells with CD45.2 + -mutant LSK cells from the same Rx291/Ezh2 Δ/Δ mice ( Fig. 5c ), but not from Rx291fs mice ( Supplementary Fig. 6 ). Indeed, Rx291/Ezh2 Δ/Δ -MDS (CD45.2 + GFP + ) LSK cells significantly upregulated IL-6, compared with WT LSK cells ( Fig. 5d ). Given that IL-6 and TNFα impair normal HSC function in vivo [43] , we examined levels of IL-6 and TNFα proteins in BM cells and circulating amount of IL-6 in PB serum. Levels of IL-6, but not TNFα, were significantly elevated in Rx291/Ezh2 Δ/Δ BM cells ( Fig. 5e ). Stimulation of BM cells with an endotoxin, lipopolysaccharide (LPS), for 5 h ex vivo , increased the amount of not only IL-6 but also TNFα to levels significantly higher in Rx291/Ezh2 Δ/Δ BM cells compared with Rx291 BM cells ( Fig. 5e ). In addition, Rx291/Ezh2 Δ/Δ mice at the MDS stage showed significantly elevated levels of circulating IL-6 protein in the PB serum ( Fig. 5f ). These findings indicate that Rx291/Ezh2 Δ/Δ -MDS cells, despite their compromised proliferative capacity, outcompete WT HSPCs by impeding their function via an inflammation-related mechanism in the MDS BM environment. 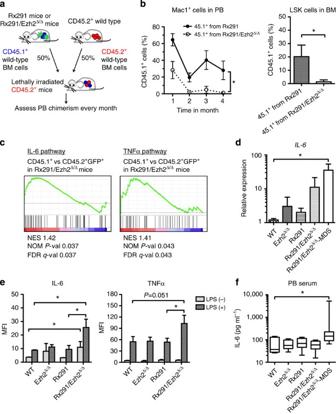Figure 5: Impaired normal HSPC functions in RUNX1S291fs/Ezh2-null mice. (a) Experimental scheme of analysing function of CD45.1+WT BM cells in Rx291 mice and Rx291/Ezh2Δ/Δmice. CD45.1+WT (2 × 105) BM cells isolated from Rx291 and Rx291/Ezh2Δ/Δmice were transplanted into lethally irradiated CD45.2+mice along with the same number of freshly isolated CD45.2+WT (2 × 105) BM cells. (b) Repopulation capacity of CD45.1+WT cells from Rx291 and Rx291/Ezh2Δ/Δmice. Chimerism of CD45.1+Mac1+myeloid cells in PB (left panel) and LSK cells (right panel) in BM at 4 months post transplantation is depicted (n=3). Scale bars and asterisk show mean±s.d. and *P<0.05 by Student’st-test. (c) Gene set enrichment plots for IL-6 (ref. 54)54(left panel) and TNFα (TNF receptor signalling, Pathway Interaction Database)(right panel) pathway gene sets comparing CD45.1+WT LSK cells to CD45.2+GFP+mutant LSK cells in Rx291/Ezh2Δ/Δmice. (d) Quantitative RT–PCR analysis of the expression ofIL-6in CD45.2+GFP+LSK cells from WT, Ezh2Δ/Δ, Rx291 and Rx291/Ezh2Δ/Δmice at 4 months post transplantation (pre-MDS stage) and from moribund Rx291/Ezh2Δ/Δ-MDS mice (n=4–5). Scale bars and asterisk show mean±s.d. and *P<0.05 by Mann–WhitneyU-test. (e) Levels of IL-6 and TNFα proteins in CD45.2+GFP+BM cells from WT, Ezh2Δ/Δ, Rx291 and Rx291/Ezh2Δ/Δmice (at pre-MDS stage) (n=3–6) when cultured with or without 10 ng ml−1LPS for 5 hoursin vitro. Expression levels were examined by flow cytometry and shown in mean fluorescence intensity (MFI). Scale bars and asterisk show means±s.e.m and *P<0.05 by Student’st-test. (f) Levels of IL-6 protein in the PB serum from WT, Ezh2Δ/Δ, Rx291 and Rx291/Ezh2Δ/Δmice (at pre-MDS stage) and from moribund Rx291/Ezh2Δ/Δ-MDS mice (n=6–8). Expression levels were examined by enzyme-linked immunosorbent assay utilizing anti-IL-6 antibody and are shown as box and whisker plots, *P<0.05 by Mann–WhitneyU-test. Figure 5: Impaired normal HSPC functions in RUNX1S291fs/Ezh2-null mice. ( a ) Experimental scheme of analysing function of CD45.1 + WT BM cells in Rx291 mice and Rx291/Ezh2 Δ/Δ mice. CD45.1 + WT (2 × 10 5 ) BM cells isolated from Rx291 and Rx291/Ezh2 Δ/Δ mice were transplanted into lethally irradiated CD45.2 + mice along with the same number of freshly isolated CD45.2 + WT (2 × 10 5 ) BM cells. ( b ) Repopulation capacity of CD45.1 + WT cells from Rx291 and Rx291/Ezh2 Δ/Δ mice. Chimerism of CD45.1 + Mac1 + myeloid cells in PB (left panel) and LSK cells (right panel) in BM at 4 months post transplantation is depicted ( n =3). Scale bars and asterisk show mean±s.d. and * P <0.05 by Student’s t -test. ( c ) Gene set enrichment plots for IL-6 (ref. 54) [54] (left panel) and TNFα (TNF receptor signalling, Pathway Interaction Database)(right panel) pathway gene sets comparing CD45.1 + WT LSK cells to CD45.2 + GFP + mutant LSK cells in Rx291/Ezh2 Δ/Δ mice. ( d ) Quantitative RT–PCR analysis of the expression of IL-6 in CD45.2 + GFP + LSK cells from WT, Ezh2 Δ/Δ , Rx291 and Rx291/Ezh2 Δ/Δ mice at 4 months post transplantation (pre-MDS stage) and from moribund Rx291/Ezh2 Δ/Δ -MDS mice ( n =4–5). Scale bars and asterisk show mean±s.d. and * P <0.05 by Mann–Whitney U -test. ( e ) Levels of IL-6 and TNFα proteins in CD45.2 + GFP + BM cells from WT, Ezh2 Δ/Δ , Rx291 and Rx291/Ezh2 Δ/Δ mice (at pre-MDS stage) ( n =3–6) when cultured with or without 10 ng ml −1 LPS for 5 hours in vitro . Expression levels were examined by flow cytometry and shown in mean fluorescence intensity (MFI). Scale bars and asterisk show means±s.e.m and * P <0.05 by Student’s t -test. ( f ) Levels of IL-6 protein in the PB serum from WT, Ezh2 Δ/Δ , Rx291 and Rx291/Ezh2 Δ/Δ mice (at pre-MDS stage) and from moribund Rx291/Ezh2 Δ/Δ -MDS mice ( n =6–8). Expression levels were examined by enzyme-linked immunosorbent assay utilizing anti-IL-6 antibody and are shown as box and whisker plots, * P <0.05 by Mann–Whitney U -test. Full size image RUNX1S291fs helps PRC1 repress Hoxa9 in the absence of Ezh2 MDS patients with EZH2 mutations show low risk of transformation to AML and EZH2 mutations are rare in de novo AML [2] . Indeed, none of the Rx291/Ezh2 Δ/Δ mice developed typical de novo AML in this study. We therefore examined expression of target genes of MLL-AF9 and NUP98-HOXA9 fusions [44] , [45] in LSK cells by GSEA, and found that Rx291/Ezh2 Δ/Δ -MDS LSK cells had negative enrichment of canonical AML target genes ( Table 2 and Supplementary Fig. 7 ). Among these AML target genes, Hoxa9 is critical for both HSCs and MLL-AF9 -positive AML cells [44] , [46] . Expression of Hoxa9 was downregulated in LSK cells expressing RUNX1S291fs mutant and further depressed by Ezh2 loss at the MDS stage ( Fig. 6a ). RT–PCR confirmed that expression of Hoxa9 as well as that of Hoxa10 , another oncogene characteristic of AML, was significantly downregulated in Rx291/Ezh2 Δ/Δ -MDS LSK cells compared with WT LSK cells ( Fig. 6b ). 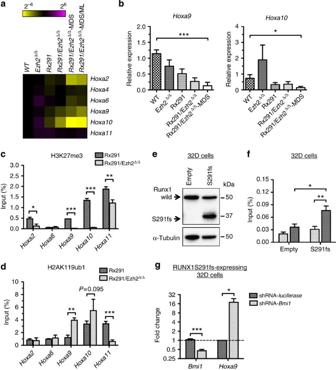Figure 6: RUNX1S291fs helps PRC1 repressHoxa9expression in the absence of Ezh2. (a) Heat map showing expression profiles ofHoxagenes in CD45.2+GFP+LSK cells from WT, Ezh2Δ/Δ, Rx291 and Rx291/Ezh2Δ/Δmice at 4 months post transplantation (pre-MDS stage) and from moribund Rx291/Ezh2Δ/Δ-MDS and MDS/ML mice. (b) Quantitative RT–PCR analysis of the expression ofHoxa9andHoxa10in LSK cells from WT, Ezh2Δ/Δ, Rx291 and Rx291/Ezh2Δ/Δmice at 4 months post transplantation (pre-MDS stage) and from moribund Rx291/Ezh2Δ/Δ-MDS mice (n=4–5). Scale bars and asterisk show mean±s.d., *P<0.05 and ***P<0.001 by Student’st-test. (c,d) Levels of H3K27me3 (c) and H2AK119ub1 (d) at the promoters ofHoxagenes inRx291andRx291/Ezh2Δ/ΔLSK cells as detected by ChIP–QPCR. The relative amounts of immunoprecipitated DNA are depicted as a percentage of input DNA. Scale bars and asterisks show mean±s.e.m., *P<0.05, **P<0.01 and ***P<0.001 by Student’st-test (n=4). (e) Detection of RUNX1S291fs protein inRUNX1S291fs-expressing 32D cells by western blotting using an anti-RUNX1 antibody. α-Tubulin was detected as a loading control. Arrows indicate endogenous Runx1 and RUNX1S291fs proteins. (f) Recruitment of Bmi1 to theHoxa9promoter inRUNX1S291fs-expressing 32D cells. Localization of Bmi1 at theHox9apromoter was evaluated in 32D cells andRUNX1S291fs-expressing 32D cells by ChIP–QPCR. The relative amounts of immunoprecipitated DNA are depicted as a percentage of input DNA. Scale bars and asterisks show means±s.e.m., *P<0.05 and **P<0.01 by Student’st-test (n=3). (g) Derepression ofHoxa9by knockdown ofBmi1detected by quantitative RT–PCR. 32D cells expressing RUNX1S291fs were infected with lentiviruses expressing shRNA directed to aLuciferasecontrol orBmi1. Scale bars and asterisk show mean±s.e.m., *P<0.05 and ***P<0.001 by Student’st-test (n=4). Figure 6: RUNX1S291fs helps PRC1 repress Hoxa9 expression in the absence of Ezh2. ( a ) Heat map showing expression profiles of Hoxa genes in CD45.2 + GFP + LSK cells from WT, Ezh2 Δ/Δ , Rx291 and Rx291/Ezh2 Δ/Δ mice at 4 months post transplantation (pre-MDS stage) and from moribund Rx291/Ezh2 Δ/Δ -MDS and MDS/ML mice. ( b ) Quantitative RT–PCR analysis of the expression of Hoxa9 and Hoxa10 in LSK cells from WT, Ezh2 Δ/Δ , Rx291 and Rx291/Ezh2 Δ/Δ mice at 4 months post transplantation (pre-MDS stage) and from moribund Rx291/Ezh2 Δ/Δ -MDS mice ( n =4–5). Scale bars and asterisk show mean±s.d., * P <0.05 and *** P <0.001 by Student’s t -test. ( c , d ) Levels of H3K27me3 ( c ) and H2AK119ub1 ( d ) at the promoters of Hoxa genes in Rx291 and Rx291/Ezh2 Δ/Δ LSK cells as detected by ChIP–QPCR. The relative amounts of immunoprecipitated DNA are depicted as a percentage of input DNA. Scale bars and asterisks show mean±s.e.m., * P <0.05, ** P <0.01 and *** P <0.001 by Student’s t -test ( n =4). ( e ) Detection of RUNX1S291fs protein in RUNX1S291fs -expressing 32D cells by western blotting using an anti-RUNX1 antibody. α-Tubulin was detected as a loading control. Arrows indicate endogenous Runx1 and RUNX1S291fs proteins. ( f ) Recruitment of Bmi1 to the Hoxa9 promoter in RUNX1S291fs -expressing 32D cells. Localization of Bmi1 at the Hox9a promoter was evaluated in 32D cells and RUNX1S291fs -expressing 32D cells by ChIP–QPCR. The relative amounts of immunoprecipitated DNA are depicted as a percentage of input DNA. Scale bars and asterisks show means±s.e.m., * P <0.05 and ** P <0.01 by Student’s t -test ( n =3). ( g ) Derepression of Hoxa9 by knockdown of Bmi1 detected by quantitative RT–PCR. 32D cells expressing RUNX1S291fs were infected with lentiviruses expressing shRNA directed to a Luciferase control or Bmi1 . Scale bars and asterisk show mean±s.e.m., * P <0.05 and *** P <0.001 by Student’s t -test ( n =4). Full size image In contrast to Mecom/Evi1 , promoter DNA hypermethylation was not involved in the repression of Hoxa9 expression in Rx291/Ezh2 Δ/Δ LSK cells ( Supplementary Fig. 8 ). We and other group recently reported that RUNX1 recruit PRC1 via direct binding to Bmi1 to establish transcriptional repression of genes in a context-dependent manner [12] , [47] . We therefore hypothesized that the RUNX1S291fs mutant might collaborate with Bmi1 to suppress expression of Hoxa9. We first performed a chromatin immunoprecipitation (ChIP)–QPCR assay for H3K27me3 and H2AK119ub1 at promoters of the Hoxa gene cluster using Rx291 and Rx291/Ezh2 Δ/Δ LSK cells. We found that levels of H3K27me3 were markedly reduced at Hoxa9 and Hoxa10 promoters in Rx291/Ezh2 Δ/Δ cells ( Fig. 6c ). By contrast, H2AK119ub1 was significantly enriched at the Hoxa9 promoter in Rx291/Ezh2 Δ/Δ cells compared with Rx291 cells ( Fig. 6d ). To determine whether Bmi1 binds to the promoter region of Hoxa9 , we performed a ChIP–QPCR assay using an anti-Bmi1 antibody in murine 32D cells expressing RUNX1S291fs ( Fig. 6e ) due to the paucity of primary LSK cells. As expected, Bmi1 significantly bound to the Hoxa9 promoter in RUNX1S291fs-expressing 32D cells compared with the control 32D cells ( Fig. 6f ). To determine whether the recruitment of Bmi1 contributed to transcriptional repression of Hoxa9 , we transduced short hairpin RNA (shRNA) directed to Bmi1 or luciferase , a negative control, in RUNX1S291fs -expressing 32D cells. Knockdown of Bmi1 induced a significant elevation of Hoxa9 expression in RUNX1S291fs -expressing 32D cells ( Fig. 6g ). We also observed that RUNX1S291fs mutant physically associates with Bmi1 in RUNX1S291fs-expressing 32D cells ( Supplementary Fig. 9 ). Taken together, the RUNX1S291fs mutant promotes PRC1-mediated transcriptional repression of Hoxa9 in the absence of Ezh2. While Ezh2 loss alone did not significantly affect the levels of H3K27me3 at the promoter of Hoxa9 , it induced a mild increase in the levels of H2AK119ub1 and moderately repressed the expression of Hoxa9 ( Fig. 6b and Supplementary Fig. 10 ). These findings imply that Ezh2 loss could also lead to the transcriptional repression of Hoxa9 , although the underlying mechanism is obscure. Inactivation of Hoxa9 restrains MDS from leukaemic formation We next interrogated the pathophysiological relevance of reduced Hoxa9 expression to MDS. We first examined expression of HOXA9 in CD34 + stem/progenitor cells isolated from RCMD (refractory cytopenia with multilineage dysplasia), RAEBI/II (refractory anaemia with excess blasts I/II), MDS/AML, de novo AML patients and healthy volunteers by quantitative RT–PCR. While the level of HOXA9 expression in MDS–RCMD and de novo AML patients was comparable to the control CD34 + cells, it was significantly elevated to the levels higher than those of MLL-AF9 -positive AML cell lines in both MDS–RAEBI/II and MDS/AML patients ( Fig. 7a ). Thus, HOXA9 expression is robustly activated in high-risk MDS and MDS/AML patients, suggesting that the level of HOXA9 expression is critical to the leukaemic transformation of MDS. 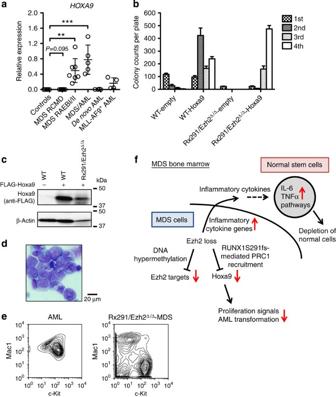Figure 7:Hoxa9expression level is critical for transformation from MDS to AML. (a) Quantitative RT–PCR analysis of the expression ofHOXA9in CD34+cells of seven MDS–RCMD, seven MDS–RAEBI/II, five MDS/AML, fourde novoAML patients, fourMLL-AF9-positive AML cell lines (THP-1, NOMO-1, MOLM-13 and MONO-MAC1) and six healthy controls. Scale bars and asterisks show mean±s.d., **P<0.01, and ***P<0.001 by Mann–WhitneyU-test. (b,c) Clonogenic capacity ofRx291/Ezh2Δ/Δcells overexpressingHoxa9. WT andRx291/Ezh2Δ/ΔHSCs were transduced with aHoxa9retrovirus and plated in methylcellulose media, then replated into the same medium every 14 days. The data are shown as mean±s.e.m. (n=3) inb. Expression of exogenous Flag-tagged Hoxa9 protein in colony cells was detected by western blotting using an anti-Flag antibody inc. β-Actin was detected as a loading control. (d) Morphology of AML cells from BM of recipients infused withHoxa9-expressingRx291/Ezh2Δ/Δcells observed by May–Grüenwald Giemsa staining. Scale bar, 20 μm. (e) Fluorescence-activated cell sorting profiles of BM cells from mouse indand Rx291/Ezh2Δ/Δ-MDS mouse. (f) A proposed model of the role of Ezh2 loss in the development ofRUNX1S291fs-induced MDS. Figure 7: Hoxa9 expression level is critical for transformation from MDS to AML. ( a ) Quantitative RT–PCR analysis of the expression of HOXA9 in CD34 + cells of seven MDS–RCMD, seven MDS–RAEBI/II, five MDS/AML, four de novo AML patients, four MLL-AF9 -positive AML cell lines (THP-1, NOMO-1, MOLM-13 and MONO-MAC1) and six healthy controls. Scale bars and asterisks show mean±s.d., ** P <0.01, and *** P <0.001 by Mann–Whitney U -test. ( b , c ) Clonogenic capacity of Rx291/Ezh2 Δ/Δ cells overexpressing Hoxa9 . WT and Rx291/Ezh2 Δ/Δ HSCs were transduced with a Hoxa9 retrovirus and plated in methylcellulose media, then replated into the same medium every 14 days. The data are shown as mean±s.e.m. ( n =3) in b . Expression of exogenous Flag-tagged Hoxa9 protein in colony cells was detected by western blotting using an anti-Flag antibody in c . β-Actin was detected as a loading control. ( d ) Morphology of AML cells from BM of recipients infused with Hoxa9 -expressing Rx291/Ezh2 Δ/Δ cells observed by May–Grüenwald Giemsa staining. Scale bar, 20 μm. ( e ) Fluorescence-activated cell sorting profiles of BM cells from mouse in d and Rx291/Ezh2 Δ/Δ -MDS mouse. ( f ) A proposed model of the role of Ezh2 loss in the development of RUNX1S291fs -induced MDS. Full size image To test this hypothesis, we transduced ectopic Hoxa9 into HSCs from WT and Rx291/Ezh2 Δ/Δ mice. To evaluate the proliferative capacity of Hoxa9 -expressing Rx291/Ezh2 Δ/Δ HSCs, we first conducted serial replating assays in vitro . While Rx291/Ezh2 Δ/Δ cells did not form colonies after the second plating, Hoxa9 -expressing Rx291/Ezh2 Δ/Δ cells acquired the capability to give rise to colonies and efficiently generated colonies even after the fourth replating, similar to Hoxa9 -expressing WT cells ( Figs 7b,c ). We next transplanted Hoxa9 -expressing HSCs into lethally irradiated recipient mice together with life-saving 2 × 10 5 BM cells. Notably, two out of four recipients transplanted with Hoxa9 -expressing Rx291/Ezh2 Δ/Δ cells developed AML with increased myeloblast cells ( Fig. 7d ), and died by 6 months post transplantation, while Hoxa9 -expressing WT cells developed neither MPN nor AML within the observation period, possibly due to a longer latency [48] . Hoxa9 -expressing Rx291/Ezh2 Δ/Δ AML cells in the BM highly expressed both Mac1 and c-Kit antigens ( Fig. 7e ), similar to MLL-AF9 -induced AML cells [15] . This phenotype was clearly distinct from Rx291/Ezh2 Δ/Δ -MDS cells in the BM ( Fig. 7e ). Taken together, the repressed Hoxa9 expression inhibits the leukaemic transformation of Rx291/Ezh2 Δ/Δ -MDS cells. Our studies show that the loss of Ezh2 promotes initiation and propagation of RUNX1 mutant-induced MDS, which supports a tumour-suppressive role for EZH2 in MDS. Our mouse model with concurrent Ezh2 loss and RUNX1S291fs expression developed MDS-like features such as anaemia, leukopenia, impaired myeloid cells differentiation and multilineage dysplasia. In addition, our mouse model showed an obvious resistance to transform into AML as reported that a few de novo AML patients show mutations of EZH2 (refs 1 , 2 , 18 ). Indeed, our MDS mice showed a gene expression profile distinct from AML induced by MLL-AF9 or NUP98-HOXA9 (refs 44 , 45 ). Interestingly, expression of Hoxa9 , one of the most well-known leukaemic oncogenes, was dramatically repressed in our MDS mice in contrast to AML. It has been reported that Hoxa9 deficiency impairs the proliferative capacity of HSCs, delays myeloid cell differentiation and decreases neutrophil counts [46] , a phenotype that is quite similar to the ineffective hematopoiesis observed in Rx291/Ezh2 Δ/Δ -MDS mice, except for the dysplasia we observed. Although it remains unknown how downregulation of Hoxa9 contributes to the development of MDS, we found that level of HOXA9 expression in human CD34 + cells was clearly correlated with the disease progression of MDS in patients. Given that AML transformation was induced by the ectopic expression of Hoxa9 in Rx291/Ezh2 Δ/Δ cells, we propose that the resistance to AML transformation in the absence of Ezh2 is at least in part dependent on the repression of Hoxa9 expression. Another prototypical HSC regulator that has also been shown to drive leukaemia is MECOM/EVI1 (ref. 39 ). In line with our observations in this study, however, expression of EVI1 is generally low in MDS patients [47] . Downregulation of Mecom/Evi1 expression may also contribute to the resistance to AML transformation in the absence of Ezh2. These findings indicate that our mouse model utilizing Ezh2 loss and the RUNX1S291fs mutant accurately recapitulates many aspects of MDS harbouring EZH2 mutations. In MDS patients, mutant cells propagate in the BM despite impaired proliferative capacity and are thought to eventually outcompete normal hematopoietic cells [35] . Our findings in Rx291/Ezh2 Δ/Δ -MDS mice provided a clue to understand the mechanism of clonal competition between MDS clones and normal cells in MDS patients. Rx291/Ezh2 Δ/Δ -MDS cells appeared to be defective in proliferative capacity as evidenced by the reduced expression of two potent leukaemic oncogenes, Hoxa9 and Mecom/Evi1 . Of interest, inflammatory cytokine pathways such as IL-6 pathway, which are inhibitory towards HSCs [42] were significantly activated in residing normal HSPCs, but not in Rx291/Ezh2 Δ/Δ -mutant HSPCs in the same Rx291/Ezh2 Δ/Δ mice. Indeed, expression of IL-6 was significantly elevated in Rx291/Ezh2 Δ/Δ BM cells compared with Rx291 BM cells at the level of both transcript and protein. Rx291/Ezh2 Δ/Δ BM cells exhibited heightened sensitivity to LPS stimulation, and the level of circulating IL-6 protein in the PB serum was significantly elevated in Rx291/Ezh2 Δ/Δ mice during the development of MDS. Excessive IL-6 production by MDS cells has also been shown to promote leukopenia and thrombocytosis through the activation of Traf6 in a 5q-MDS mouse model [49] . In addition, combined exposure of IL-6, CCL2 and TNFα has been reported to impair normal HSC function in vivo and inhibition of these cytokines rescues the impaired HSC function [43] . Recent studies indicated that CML cells alter the BM microenvironment to impair normal HSCs, but favour CML stem cells function, at least in part, via activation of inflammatory cytokines [29] , [30] . All these findings support that activation of inflammatory cytokine responses largely accounts for compromised normal hematopoiesis in our MDS model. In our model, Rx291/Ezh2 Δ/Δ -MDS cells outcompete normal cells by activating inflammatory responses, thereby achieving clonal expansion despite their compromised proliferative capacity ( Fig. 7f ). Our findings provide additional evidence of non-autonomous cells mechanisms that promote the expansion of MDS clones in the MDS BM environment. Since Ezh2 functions to repress transcription via H3K27me3 modification, its absence could lead to the activation of its target genes [7] . However, we observed that Ezh2 target genes were mostly kept transcriptionally repressed in Rx291/Ezh2 Δ/Δ HSPCs at the MDS stage. We have recently shown that Tet2 KD/KD Ezh2 Δ/Δ MDS LSK cells maintain the transcriptional repression of Ezh2 targets via the complementary function of Ezh1 (ref. 20) [20] . Similarly, we observed residual enrichments of H3K27me3 at specific genes (for example, Hoxa11 ), so the same mechanism may also operate in RUNX1S291fs/Ezh2 -null MDS cells. In this study, however, we identified two alternative epigenetic mechanisms underlying the repression of Ezh2 targets in RUNX1S291fs -expressing cells ( Fig. 7f ). First, Rx291/Ezh2 Δ/Δ HSPCs showed promoter DNA hypermethylation at some Ezh2 target genes, and this appeared to repress expression of important developmental regulator genes of both hematopoietic and non-hematopoietic lineages (for example, Mecom/Evi1 , Pdx1 and Hand1 ). As described above, expression of MECOM/EVI1 is generally low in MDS patients and its upregulation may trigger leukaemic transformation [24] , [47] Our findings raise the possibility that promoter DNA hypermethylation is a major molecular mechanism that keeps MECOM/EVI1 transcriptionally repressed in MDS patients. Second, we found that expression of Hoxa9 was repressed through RUNX1S291fs-directed PRC1 recruitment in the absence of Ezh2. Importantly, HOXA9 expression is closely repressed in MDS–RCMD patients irrespective of the RUNX1 mutations. Given that repression of Hoxa9 is critical to attenuate the predisposition of MDS to develop into AML, there are presumably several different ways to establish repression of Hoxa9 , and it would be intriguing to address this issue. Nonetheless, the repressed Hoxa9 expression appears to be a hallmark of MDS-specific epigenetic alteration. In conclusion, our findings provide a comprehensive picture of how Ezh2 loss functions to collaborate with RUNX1 mutant in the pathogenesis of MDS in both cell autonomous and non-autonomous manners, and how it attenuates the predisposition of MDS clones to transform into AML. While many studies have demonstrated that EZH2 functions as an oncogene in various tumours, we have experimentally demonstrated the tumour-suppressive function of EZH2 in MDS in vivo . Since there are only a few mouse models available for human MDS [34] , we hope that this MDS model will contribute to our understanding of the role of altered epigenetic regulations in the pathogenesis of MDS and to the innovation of novel therapies for MDS. Mice Ezh2 conditional knockout ( Ezh2 flox/flox ) mice were previously described, and crossed with Rosa26-Cre-ERT mice for conditional deletion [32] . C57BL/6 mice congenic for the Ly5 locus (CD45.1) were purchased from Sankyo-Lab Service. All experiments using the mice were performed in accordance with our institutional guidelines for the use of laboratory animals and approved by the Review Board for animal experiments of Chiba University (approval ID: 25-104) or Cincinnati Children's Hospital Medical Center. Retroviral transduction and transplantation pMYs-empty control-IRES-GFP , pMYs-RUNX1S291fs-IRES-GFP and pMYs-RUNX1D171N-IRES-GFP vectors were previously described [24] . CS-H1-shRNA-EF-1α-EGFP vector expressing shRNA-directed Bmi1 or luciferase were previously described [50] . Hoxa9 cDNA was kindly provided by Dr Takuro Nakamura, and the cDNA was subcloned into pMYs vector. Retrovirus infection into CD34 − LSK HSCs was performed as previously described [51] . Briefly, retrovirus-infected 50 HSCs were cultured in SF-O3 medium containing 50 ng ml −1 mouse SCF and 50 ng ml −1 human TPO for 3 days, and then these HSCs were intravenously injected in 8.5 Gy or 9 Gy irradiated CD45.1 + mice together with radioprotective 2 × 10 5 CD45.1 + BM cells. At 6 weeks post transplantation, 1 mg tamoxifen was administered via intraperitoneal injection for 5 consecutive days to completely delete Ezh2 alleles [32] . Colony assay Colony assays were performed in Methocult M3234 (Stem Cell Technologies) supplemented with 20 ng ml −1 mouse SCF, 20 ng ml −1 mouse IL-3, 20 ng ml −1 human TPO and 2 units ml −1 human EPO. The number of colonies was counted at day14 of culture. For replating assay, colonies were scored at day14 and pooled 3 × 10 4 cells were replated into the same medium. Cell culture BM cells were stimulated with or without 10 ng ml −1 LPS ( Escherichia coli 0127:B8; Sigma-Aldrich) in 10% fetal bovine serum RPMI supplemented with 10 ng ml −1 mouse IL-3 and GolgiStop (BD 554724) containing monensin, which inhibits intracellular protein transport processes. Flow cytometry and antibodies Flow cytometry and cell sorting were performed by utilizing the following monoclonal antibodies; CD45.2 (104), CD45.1 (A20), Gr1 (RB6-8C5), CD11b/Mac1 (M1/70), Ter119, CD71 (R17217), CD127/IL-7Rα (A7R34), B220 (RA3-6B2), CD4 (L3T4), CD8α (53-6.7), CD117/c-Kit (2B8), Sca1 (D7), CD34 (MEC14.7) and FcγRII-III (93) [32] . These antibodies were purchased from eBioscience or BioLegend. Lineage mixture solution contains Gr1, Mac1, B220, CD4, CD8α, Ter119 and IL-7Rα biotin-conjugated antibodies. Apoptotic cells were stained with anti-Annexin V-APC antibody (BD 550474) and with propidium iodide following staining cell surface markers to discriminate Lineage − Sca1 + c-Kit + cells or CD71 + Ter119 + cells. To evaluate cellular proliferation, cells were fixed and permeabilized (FIX & PERM, Invitrogen) according to the manufacturer’s instruction, and then detected by using anti-Ki67-PE antibody (BD 556027) following staining cells by lineage mixture, streptavidin-APC-Cy7, Sca1 PE-Cy7 and c-Kit APC antibodies. To evaluate intracellular amounts of IL-6 and TNFα proteins, BM cells were fixed and permeabilized and then detected by using anti-IL-6 (BD 554401) and anti-TNFα (BD 557730) antibodies following staining cells with CD45.2 antibody. All flow cytometry analyses and cell sorting were performed on FACSAriaII or FACSCantoII (BD). Quantitative RT–PCR Quantitative RT–PCR was performed on a StepOnePlus Real time PCR System (Life Technologies) by using SYBR Premix Ex TaqII (Takara) or FastStart Universal Probe Master (Roche) with a Universal Probe Library (Roche) and primers shown in Supplementary Table 4 . The expression levels of HOXA9 and GAPDH were examined by using TaqMan Gene Expression Assays (Hs03929097_g1 and Hs00266821_m1, respectively; Life Technologies). All data are presented as relative expression levels normalized to either Gapdh or GAPDH expression. Microarray analysis Total RNA was extracted from ~\n2 × 10 5 pooled BM LSK cells (isolated from two to four mice per each genotype except diseased mouse) by using an RNeasy Plus Mini Kit (Qiagen). A quantity of 20 ng of total RNA was mixed with spike-in controls using an Agilent One Colour Spike Mix Kit (Agilent), amplified and labelled with Cyanine 3 using a Low Input Quick Amp Labeling Kit (Agilent) according to the manufacturer's instructions. Microarray analysis using a SurePrint G3 Mouse GE Microarray 8 × 60 K kit (Agilent) was performed according to the manufacturer's instructions. The raw data were deposited in Gene Expression Omnibus under the accession number GSE50537. Western blotting ChIP and quantitative RT–PCR Antibodies for western blotting and immunoprecipitation were as follows: anti-H3 (Abcam, ab1791), anti-H3K27me3 (Millipore 07449), anti-Bmi1 (clone 8A9, kindly provided by Dr N. Nozaki, MAB Institute), anit-RUNX1 (Abcam, ab23980), anti-FLAG (M2, Sigma), anti-β-Actin (Santa Cruz, sc-47778), and anti-α-Tubulin (Santa Cruz, sc-5286). Uncropped raw scans of blots used in the figures are presented in Supplementary Fig. 11 . ChIP assays were performed as previously described [15] . Briefly, 1 × 10 5 pooled BM LSK cells were used for each immunoprecipitation. The following antibodies were used for the immunoprecipitation reactions: anti-H3K27me3 (Millipore 07449), anti-H2AK119ub1 (Cell Signaling, 8240), anti-Bmi1 (Bethyl A301694A) and pre-immune immunoglobulin G. DNA was amplified by quantitative RT–PCR on a StepOnePlus Real time PCR System (Life Technologies) using primers shown in Supplementary Table 4 . Cytokine assay Amounts of mouse IL-6 in PB serum were measured by ELISA kit (BD Bioscience) according to the manufacturer’s protocol. RRBS Total 500 ng genomic DNA extracted from LSK cells (isolated from two to three mice per each genotype and a disease mouse) were digested with MspI restriction enzyme that recognizes and cleaves CCGG tetranucleotide sequences irrespective of their methylation. DNA fragments were then subjected to end-repair and dA-tailing using an NEBNext DNA Library Prep Master Mix Set (NEB, Ipswich, MA), followed by the ligation with methylated adaptor oligo-DNA (Illumina, San Diego, CA). After the bisulphite conversion from unmethylated cytosine to uracil by using an EZ DNA Methylation kit (Zymo Research, Irvine, CA) followed by agarose gel excision of fragments ranging from 150 bp to 400 bp, DNA fragments ligated with adaptors in both ends were amplified by 18 cycles of PCR using PE1.0 and PE2.0 oligo primers (Illumina). The generated library was sequenced by the 36 bp single-end protocol of GAIIx (Illumina) using two lanes of a flow cell. As unmethylated cytosine of the library is converted to thymine during the PCR amplification, mapping of sequenced tags to murine reference genome (mm9, UCSC Genome Browser) was performed by Bismark software [52] , which can align bisulphite-converted tags to genome and evaluate their methylation simultaneously. In this study, methylation level was estimated in CpGs with ≥10 reads (713,353 CpGs per sample in an average). Statistical analysis was done by methyl kit [53] . As promoters were defined as regions spanning −2.5 to +0.5 Kb from transcription start sites and containing ≥5 CpGs that can be evaluated as ≥10 reads, these promoter regions were taken into account for differential methylation analysis. The raw data were deposited in DDBJ under the accession numbers, DRA001143, DRA001144, DRA001145 and DRA001146. MDS patient samples This study comprises MDS–RCMD ( n =7), MDS–RAEBI/II ( n =7), MDS/AML ( n =5) and de novo AML ( n =4) patients at the Hiroshima University Hospital. CD34 + blood cells were isolated using a CD34 MicroBead kit and autoMACS system (Milteny Biotec, Germany). Patient anonymity was ensured, and the study was approved by the Institutional Review Committee at Hiroshima University. Patients gave written informed consent for the study according to the Declaration of Helsinki. Accession codes : The microarray data has been deposited in the Gene Expression Omnibus under accession code GSE50537 . The bisulphite sequencing data have been deposited in the DDBJ under the accession codes DRA001143 , DRA001144 , DRA001145 and DRA001146 . How to cite this article: Sashida, G. et al. Ezh2 loss promotes development of myelodysplastic syndrome but attenuates its predisposition to leukaemic transformation. Nat. Commun. 5:4177 doi: 10.1038/ncomms5177 (2014).